The mitochondrial uniporter controls fight or flight heart rate increases Heart rate increases are a fundamental adaptation to physiological stress, while inappropriate heart rate increases are resistant to current therapies. However, the metabolic mechanisms driving heart rate acceleration in cardiac pacemaker cells remain incompletely understood. The mitochondrial calcium uniporter (MCU) facilitates calcium entry into the mitochondrial matrix to stimulate metabolism. We developed mice with myocardial MCU inhibition by transgenic expression of a dominant-negative (DN) MCU. Here, we show that DN-MCU mice had normal resting heart rates but were incapable of physiological fight or flight heart rate acceleration. We found that MCU function was essential for rapidly increasing mitochondrial calcium in pacemaker cells and that MCU-enhanced oxidative phoshorylation was required to accelerate reloading of an intracellular calcium compartment before each heartbeat. Our findings show that MCU is necessary for complete physiological heart rate acceleration and suggest that MCU inhibition could reduce inappropriate heart rate increases without affecting resting heart rate. Catecholamine agonists trigger physiological fight or flight increases in heart rate but the metabolic pathway(s) supplying adenosine triphosphate (ATP) for increasing heart rate are incompletely understood [1] , [2] . Cardiac pacemaker cells drive heart rate acceleration, at least in part, by augmenting energy-dependent flux of Ca 2+ through an intracellular, sarcoplasmic reticulum (SR), storage compartment [3] . SR Ca 2+ release triggers pacemaker cell membrane depolarization, leading to action potential initiation that triggers each heart beat [4] . Mitochondrial Ca 2+ entry through the mitochondrial Ca 2+ uniporter (MCU) can stimulate increased ATP production by enhancing the activity of dehydrogenases in the mitochondrial matrix that supply NADH for electron transport [5] , [6] . The recent discovery of the gene encoding the MCU protein Ca 2+ permeation pore [7] , [8] allowed us to test the potential role of MCU-mediated mitochondrial Ca 2+ entry as a pathway for increasing ATP production to fuel heart rate increases. We developed new tools and approaches for studying the metabolic role of the MCU in cardiac pacing, including surgical gene transfer to pacemaker cells and transgenic mice with myocardial and pacemaker cell targeted expression of a dominant-negative (DN) MCU with pore domain mutations that prevented rapid, MCU-mediated mitochondrial Ca 2+ entry. Here, we show that Ca 2+ entry through the MCU is essential for telegraphing enhanced metabolic demand to pacemaker cell mitochondria and promoting oxidative phosphorylation. We found that isoproterenol (ISO) stimulates oxidative phosphorylation by the MCU pathway in cardiac pacemaker cells to fuel the activity of the sarcoplasmic-endoplasmic reticulum Ca 2+ ATPase (SERCA2a), which is required for reloading SR Ca 2+ stores and sustaining fight or flight heart rate increases. Inhibition of mitochondrial Ca 2+ entry prevented increased oxidative phosphorylation, enhanced SERCA2a activity and physiological rate responses in cardiac pacemaker cells exposed to ISO. Dialysis of cardiac pacemaker cells with exogenous ATP rescued the fight or flight response to ISO despite MCU inhibition but ATP dialysis was ineffective after SERCA2a inhibition, by expression of a super-inhibitory phospholamban (PLN) mutant or thapsigargin, identifying SERCA2a as a critical control point downstream of MCU for heart rate increases and a preferential sink for mitochondrially-sourced ATP. Isolated hearts from wild-type mice with pacemaker-targeted DN-MCU gene therapy were resistant to rate increases by ISO. We found selectively obtunded ISO triggered rate increases in isolated pacemaker cells, in excised Langendorff-perfused hearts from wild-type mice with DN-MCU pacemaker-targeted gene therapy and in vivo in DN-MCU transgenic mice. Furthermore, DN-MCU transgenic mice showed reduced heart rates in response to spontaneous activity compared with wild-type littermate controls. In contrast to the profound loss of heart rate acceleration by MCU inhibition, unstimulated heart rates and autonomous pacemaker cell action potential firing were unaffected by the loss of MCU-mediated mitochondrial Ca 2+ entry. Our findings highlight a previously unrecognized subcellular mechanism for catecholamine-triggered heart rate increases and provide insight into a role for MCU-mediated mitochondrial Ca 2+ entry as a metabolic second messenger required for the physiological fight or flight stress response [9] . These results define the MCU as an essential activator of a metabolic pathway for heart rate control and suggest that MCU inhibition in cardiac pacemaker cells has therapeutic potential to selectively prevent excessive heart rates. The MCU mediates rate increases in pacemaker cells Isolated cardiac sinoatrial nodal (SAN) pacemaker cells spontaneously generate action potentials under basal conditions, in the absence of catecholamine stimulation. The rate of action potential initiation is increased with ISO, a catecholamine β-adrenergic receptor agonist, in a concentration-dependent manner ( Fig. 1a–d ) [10] . We found that SAN cells dialysed with Ru360 (5 μM), an MCU antagonist, had significantly reduced action potential frequency increases to ISO ( Fig. 1b,d ) compared with SAN cells without Ru360 ( Fig. 1a,d ). The inhibitory effect of Ru360 on SAN cell action potential frequency responses to ISO was reversed by co-dialysis with ATP (4 mM), a concentration present in heart cells ( Fig. 1c,d ) [11] . Co-dialysis with 1 and 2 mM ATP pipette solutions was inadequate to rescue ISO-mediated rate increases while 8 mM ATP did not result in greater rate responses than 4 mM ATP ( Supplementary Fig. 1a–c ), suggesting fight or flight SAN responses operate between an [ATP] threshold >2 and </=4 mM. In contrast, neither Ru360 nor ATP had any affect on basal SAN cell rates and ATP dialysis had no affect on SAN rate responses to ISO in the absence of Ru360 ( Supplementary Fig. 1a,b ), indicating that basal heart rate was independent of an MCU pathway and that exogenous ATP did not affect Ru360-independent cellular processes important for accelerating heart rate. We next corroborated our results with Ru360 dialysis by infecting SAN cells with adenovirus encoding a DN-MCU, containing pore domain charge reversal mutations that prevent MCU-mediated mitochondrial Ca 2+ entry ( Fig. 1e–h ) [7] , [8] . Both Ru360 and DN-MCU were similarly effective at preventing mitochondrial Ca 2+ entry ( Supplementary Fig. 2 ) and, like intracellular dialysis with Ru360, DN-MCU expression in SAN cells interfered with ISO-induced rate increases ( Fig. 1f,h ). The DN-MCU-dependent loss of the ISO rate response was rescued by co-dialysis with ATP ( Fig. 1g,h ), mirroring findings with MCU inhibition by Ru360 ( Fig. 1c,d ). Cultured SAN cells, with and without DN-MCU expression, had slower basal spontaneous rates than freshly isolated counterparts (baseline in Fig. 1d,h ) but nevertheless exhibited significant rate increases over baseline in response to ISO ( Fig. 1i,j ). We considered the possibility that the mitochondrial Na + /Ca 2+ exchanger, a MCU-independent pathway for mitochondrial Ca 2+ efflux, could also contribute to SAN rate increases [12] by testing SAN responses to CGP-37157 (1 μM), a Na + /Ca 2+ exchanger antagonist. After CGP-37157, we measured a 1.2±6.0% increase in WT SAN cells ( n =8) and 0.8±2.6% increase in DN-MCU SAN cells ( n =3, P =0.88), suggesting that the mitochondrial Na + /Ca 2+ exchanger did not affect basal heart rate. After ISO (1 μM), we measured a 79.8±5.8% ( n =4) increase from baseline rate in WT SAN cells and 32.0±11.1% increase from baseline ( n =4) rate in DN-MCU SAN cells ( P <0.01), similar to ISO-mediated increases in the absence of CGP-37157 ( Fig. 1i ). These findings suggested that the mitochondrial Na + /Ca 2+ exchanger was unlikely to participate in SAN rate responses, consistent with other recent findings [13] . The rescue of physiological responses to ISO after MCU inhibition by ATP dialysis suggested that MCU activity was an upstream event required to supply adequate ATP for increasing heart rate. 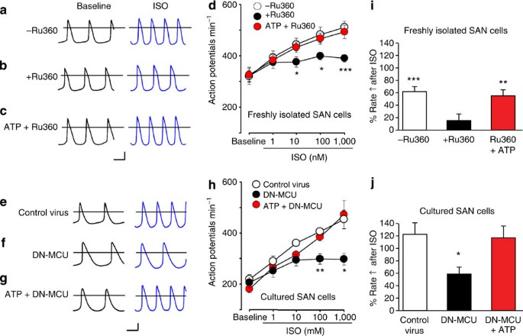Figure 1: SAN cell rate response to ISO is impaired by Ru360 or DN-MCU and rescued by ATP. (a–c) Example action potential (AP) tracings recorded under basal (left) and ISO-stimulated (right) conditions from freshly isolated SAN cells. The horizontal line marks 0 mV. Scale bars are 100 ms horizontal and 20 mV vertical. (d) Summary dose–response data for SAN cell AP rate responses to ISO. (e–g) Example AP tracings recorded under basal (left) and ISO-stimulated (right) conditions from cultured SAN cells. The horizontal line marks 0 mV. Scale bars are the same as in (a–c). (h) Summary dose–response data for cultured SAN cell AP rate responses to ISO. (i,j) Percentage rate increases over baseline after ISO in isolated SAN cells. (i) Freshly isolated SAN cells (data calculated fromd). (j) Cultured SAN cells (data calculated fromh). *P<0.05, **P<0.01, ***P<0.001, one-way analysis of variance,n=10–15 per group ind,n=5–9 per group inh.Error bars indicate s.e.m. Figure 1: SAN cell rate response to ISO is impaired by Ru360 or DN-MCU and rescued by ATP. ( a – c ) Example action potential (AP) tracings recorded under basal (left) and ISO-stimulated (right) conditions from freshly isolated SAN cells. The horizontal line marks 0 mV. Scale bars are 100 ms horizontal and 20 mV vertical. ( d ) Summary dose–response data for SAN cell AP rate responses to ISO. ( e – g ) Example AP tracings recorded under basal (left) and ISO-stimulated (right) conditions from cultured SAN cells. The horizontal line marks 0 mV. Scale bars are the same as in ( a – c ). ( h ) Summary dose–response data for cultured SAN cell AP rate responses to ISO. ( i , j ) Percentage rate increases over baseline after ISO in isolated SAN cells. ( i ) Freshly isolated SAN cells (data calculated from d ). ( j ) Cultured SAN cells (data calculated from h ). * P <0.05, ** P <0.01, *** P <0.001, one-way analysis of variance, n =10–15 per group in d , n =5–9 per group in h. Error bars indicate s.e.m. Full size image MCU inhibition impairs heart rate acceleration The selective control of pacemaker cell rate increases by MCU inhibition suggested that the MCU could be a novel target for controlling heart rate increases without slowing resting heart rates. To test this concept in hearts, we used a targeted gene-painting approach to deliver adenovirus expressing DN-MCU or eGFP to the SAN in vivo [14] . One week after SAN gene painting, we verified SAN targeted gene expression ( Fig. 2a,b ) and measured rate responses to ISO in excised, Langendorff-perfused hearts ( Fig. 2c–f ). We found DN-MCU SAN gene painting significantly and selectively reduced heart rate increases to ISO without affecting spontaneous heart rates in the absence of ISO. We next developed transgenic mice with myocardial DN-MCU expression ( Fig. 3a,b and Supplementary Fig. 3 ) to test the role of MCU in heart rate acceleration in vivo . The DN-MCU mice had hearts with normal chamber size and function ( Fig. 3c ), detectable SAN DN-MCU expression ( Fig. 3d ), reduced ATP content ( Fig. 3e ) and complete loss of mitochondrial Ca 2+ uptake in myocardial cells ( Fig. 3f,g ). DN-MCU hearts showed increased Mcu mRNA, as expected, and reduced mRNA expression for auxiliary MCU regulatory proteins ( Supplementary Fig. 4 ), possibly consistent with compensatory transcriptional reprogramming in response to the loss of functional MCU. The reduced fight or flight response in DN-MCU hearts was selective for catecholamine agonist stimulation because DN-MCU and wild-type SAN cells had similar rate responses to BayK 8644 (1 μM), a voltage-gated Ca 2+ channel agonist capable of accelerating heart rate independent of ISO. In the presence of BayK 8644 DN-MCU SAN cells ( n =5) exhibited 69.9±10.9% rate increases over baseline, similar to published responses in wild-type SAN cells [15] . During echocardiography measurements, lightly sedated DN-MCU mice exhibited resting heart rates similar to wild-type littermate controls ( Fig. 3c ). Lightly sedated and restrained DN-MCU and wild-type mice during cutaneous electrocardiogram (ECG) recording showed similar resting heart rates ( Fig. 3h–j ), but reduced ISO-stimulated heart rate increases ( Fig. 3j,k ). DN-MCU mice had significantly prolonged P-waves, PQ and PR intervals but similar QRS and QT interval durations compared with WT controls, suggesting that loss of MCU current slows atrial and atrioventricular conduction velocity without affecting conduction velocity in the distal conduction system or in ventricular myocardium ( Supplementary Table 1 ). Finally, we measured heart rates in unrestrained and unsedated mice with surgically implanted ECG and activity telemeters. DN-MCU mice showed modest but significant reductions in basal heart rate compared with wild-type controls and these differences were enhanced by activity ( Fig. 3l,m ) and ISO ( Fig. 3n,o ). Taken together, these data showed heart rate responses to spontaneous activity and ISO required MCU, whereas basal heart rates were independent of MCU, indicating MCU inhibition could selectively prevent heart rate increases in vivo . 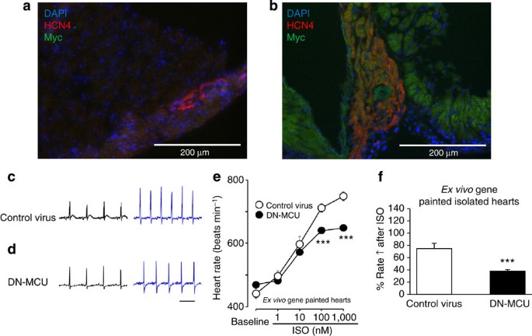Figure 2: DN-MCU gene painting impairs ISO rate response in isolated hearts. (a–b) Immunofluorescent staining of (a) control right atrium and (b) gene-painted SAN showing DAPI (blue) and HCN4 (red) to identify SAN, and Myc epitope tag (green) for DN-MCU-Myc expression. Scale bar, 200 μm. (c,d) Exampleex vivoECG tracings recorded under basal (left) and ISO-stimulated (right) conditions from gene-painted hearts. Scale bar, 100 ms. (e) Summary dose–response data forex vivoheart rate response to ISO. (f) Percentage rate increases over baseline after ISO in gene-painted isolated, Langendorff-perfused hearts (data calculated frome). ***P<0.001, unpaired Student‘st-test,n=22–24 per group ine. Error bars indicate s.e.m. Figure 2: DN-MCU gene painting impairs ISO rate response in isolated hearts. ( a – b ) Immunofluorescent staining of ( a ) control right atrium and ( b ) gene-painted SAN showing DAPI (blue) and HCN4 (red) to identify SAN, and Myc epitope tag (green) for DN-MCU-Myc expression. Scale bar, 200 μm. ( c , d ) Example ex vivo ECG tracings recorded under basal (left) and ISO-stimulated (right) conditions from gene-painted hearts. Scale bar, 100 ms. ( e ) Summary dose–response data for ex vivo heart rate response to ISO. ( f ) Percentage rate increases over baseline after ISO in gene-painted isolated, Langendorff-perfused hearts (data calculated from e ). *** P <0.001, unpaired Student‘s t -test, n =22–24 per group in e . Error bars indicate s.e.m. 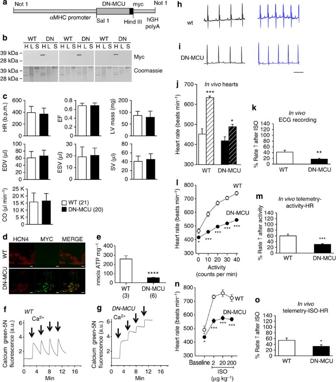Figure 3: Characterization of the DN-MCU transgenic mouse. (a) Schematic of the α-myosin heavy chain promoter-driven transgenic DN-MCU construct. (b) Western blots for Myc-tagged DN-MCU protein from heart (H), liver (L) and skeletal muscle (S) lysates (WT,n=3; DN-MCU,n=3). (c) Summary echocardiographic data showing mean±standard deviation (WT,n=21; DN-MCU,n=20). NS was identified in any parameter: heart rate (HR), ejection fraction (EF), left ventricular mass (LV mass), end diastolic volume (EDV), end systolic volume (ESV), stroke volume (SV) and cardiac output (CO). (d) Images show 10 μm sections through the SAN area. Anti-Myc (green) antibody identified cells expressing DN-MCU and the SAN was identified by anti-HCN4 enhancement (red stain). Scale bar, 50 μm. (e) Data show ATP concentrations measured in freshly isolated atrial tissue from DN-MCU and littermate WT mice. ****P<0.0001, unpaired Student‘st-test. (f,g) Representative Ca2+uptake tracings of three similar experiments in permeabilized cardiac myocytes from DN-MCU and littermate WT mice (as inSupplementary Fig. 2). Arrows represent the addition of Ca2+(100 μM). (h,i) Examplein vivoECG tracings recorded under basal (left) and ISO-stimulated (right) conditions from DN-MCU and littermate WT mice. Scale bar, 100 ms. (j) Summary data forin vivoheart rate response to ISO (10 μg kg−1). Solid bars represent baseline and hashed bars represent ISO response. *P<0.05, **P<0.01, ***P<0.001, paired Student‘st-test,n=5–6 per group, error bars indicate s.e.m. (k) Percentage rate increases over baseline after ISO inin vivoECG recordings (data calculated fromj). (l)In vivoheart rate response to activity was reduced in DN-MCU mice,n=8–11 per group. *P<0.05, **P<0.01, ***P<0.001, unpaired Student‘st-test. (m) Percentage rate increases over baseline inin vivotelemetry ECG recording with peak activity (data calculated froml). (n)In vivoheart rate response to ISO stimulation was reduced by DN-MCU expression in DN-MCU mice,n=11–28 per group. Error bars indicate s.e.m. *P<0.05, **P<0.01, ***P<0.001, unpaired Student‘st-test. (o) Percentage rate increases over baseline after ISO inin vivotelemetry ECG recording with ISO (data calculated fromn). Full size image Figure 3: Characterization of the DN-MCU transgenic mouse. ( a ) Schematic of the α-myosin heavy chain promoter-driven transgenic DN-MCU construct. ( b ) Western blots for Myc-tagged DN-MCU protein from heart (H), liver (L) and skeletal muscle (S) lysates (WT, n =3; DN-MCU, n =3). ( c ) Summary echocardiographic data showing mean±standard deviation (WT, n =21; DN-MCU, n =20). NS was identified in any parameter: heart rate (HR), ejection fraction (EF), left ventricular mass (LV mass), end diastolic volume (EDV), end systolic volume (ESV), stroke volume (SV) and cardiac output (CO). ( d ) Images show 10 μm sections through the SAN area. Anti-Myc (green) antibody identified cells expressing DN-MCU and the SAN was identified by anti-HCN4 enhancement (red stain). Scale bar, 50 μm. ( e ) Data show ATP concentrations measured in freshly isolated atrial tissue from DN-MCU and littermate WT mice. **** P <0.0001, unpaired Student‘s t -test. ( f , g ) Representative Ca 2+ uptake tracings of three similar experiments in permeabilized cardiac myocytes from DN-MCU and littermate WT mice (as in Supplementary Fig. 2 ). Arrows represent the addition of Ca 2+ (100 μM). ( h , i ) Example in vivo ECG tracings recorded under basal (left) and ISO-stimulated (right) conditions from DN-MCU and littermate WT mice. Scale bar, 100 ms. ( j ) Summary data for in vivo heart rate response to ISO (10 μg kg −1 ). Solid bars represent baseline and hashed bars represent ISO response. * P <0.05, ** P <0.01, *** P <0.001, paired Student‘s t -test, n =5–6 per group, error bars indicate s.e.m. ( k ) Percentage rate increases over baseline after ISO in in vivo ECG recordings (data calculated from j ). ( l ) In vivo heart rate response to activity was reduced in DN-MCU mice, n =8–11 per group. * P <0.05, ** P <0.01, *** P <0.001, unpaired Student‘s t -test. ( m ) Percentage rate increases over baseline in in vivo telemetry ECG recording with peak activity (data calculated from l ). ( n ) In vivo heart rate response to ISO stimulation was reduced by DN-MCU expression in DN-MCU mice, n =11–28 per group. Error bars indicate s.e.m. * P <0.05, ** P <0.01, *** P <0.001, unpaired Student‘s t -test. ( o ) Percentage rate increases over baseline after ISO in in vivo telemetry ECG recording with ISO (data calculated from n ). Full size image MCU enables rapid refilling of SR Ca 2+ in pacemaker cells Catecholamine stimulation increases heart rate by enhancing SAN cell membrane inward current and shortening the time between action potential firing [16] . Release of intracellular Ca 2+ from the SR provides the electrochemical driving force for the cell membrane Na + /Ca 2+ exchanger inward current (I NCX ) in SAN cells [17] . Elimination of SR Ca 2+ release by the toxin ryanodine or SERCA2a inhibition by thapsigargin ( Supplementary Fig. 5 ) significantly reduced the SAN response to ISO, findings that demonstrate the required connection between SR Ca 2+ release and physiological SAN cell acceleration [18] . To further test the apparent connection between MCU activity and SR Ca 2+ flux, we performed confocal line-scan measurements on SAN cells isolated from DN-MCU and wild-type control mice ( Fig. 4 ). DN-MCU SAN cells had significantly fewer diastolic Ca 2+ release events and reduced SR Ca 2+ content after ISO stimulation compared to wild-type controls, suggesting that impaired fight or flight responses by MCU inhibition occurred because of reduced SR Ca 2+ flux during physiological stress. SERCA2a activity requires ATP to pump cytoplasmic Ca 2+ to the SR lumen [19] , so we measured the rate of decay of the cytoplasmic Ca 2+ concentration ([Ca 2+ ] cyto ) using a fluorescent indicator (Fura 2 AM, 0.1 μM) to test if SERCA2a was a sink for ATP produced by an Ru360-sensitive process. ISO significantly increased the rate of decline in [Ca 2+ ] cyto compared with SAN cells in control bath solution, reflecting enhanced activity of SERCA2a ( Fig. 5a ) [20] . Ru360 dialysis slowed the decline in [Ca 2+ ] cyto after ISO ( Fig. 5b ), while co-dialysis of ATP (4 mM) with Ru360 restored the rate of [Ca 2+ ] cyto decline to ISO-stimulated values present in the absence of Ru360 ( Fig. 5c,d ). However, Ru360 did not slow the decline in [Ca 2+ ] cyto in the absence of ISO stimulation ( Fig. 5e ), consistent with the lack of effect of Ru360 on SERCA2a activity or basal SAN cell action potential frequency. In contrast to the effect of ATP dialysis on SAN cells exposed to Ru360, ATP dialysis did not significantly increase the rate of [Ca 2+ ] cyto decline ( Fig. 5f–h ) or SAN action potential frequency ( Fig. 5i ) in SAN cells isolated from mice expressing a super-inhibitory mutant form of phospholamban (N27A) [21] that constrains SERCA2a despite ISO stimulation. These results show that ISO increases SAN cell rates by actions that require MCU and SERCA2a. We considered the possibility that MCU inhibition was somehow affecting the ability of ISO to enhance phospholamban phosphorylation, which reduces the inhibitory actions of phospholamban on SERCA2a [22] . We found that atrial tissues from DN-MCU and wild-type littermates had similar increases in phospholamban phosphorylation after ISO ( Supplementary Fig. 6 ), suggesting that MCU inhibition did not interfere with SERCA2a activity by actions on phospholamban nor did DN-MCU expression promiscuously affect downstream signalling actions of ISO. We interpreted the rescue of ISO responses by exogenous ATP after the elimination of MCU-mediated Ca 2+ entry but not after SERCA2a inhibition to suggest that MCU contributes to ATP synthesis targeted for SERCA2a consumption during physiological stress. 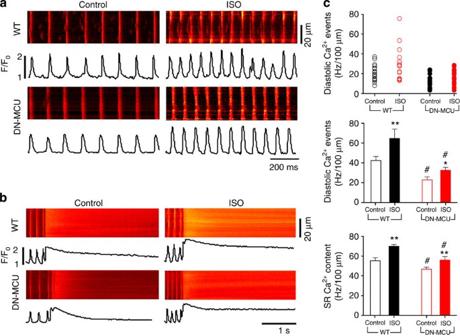Figure 4: Confocal line-scan measurements of spontaneous calcium transients and caffeine-induced calcium release in SAN cells isolated from WT and DN-MCU mice. (a) Typical calcium transient images and spatially averaged traces in spontaneous beating SAN cells. (b) Typical caffeine-induced calcium release images and spatially averaged traces. (c) Summaries of spontaneous diastolic calcium release events and SR calcium content before and after ISO. Scatter graph of diastolic calcium events before and after ISO (upper panel). Bar graph of diastolic calcium release events before and after ISO (middle panel). Bar graph of SR calcium content determined by caffeine-evoked calcium release before and after ISO (lower panel). *P<0.05, **P<0.01 versus control,#P<0.05 versus WT by Student’st-test,n=11–21 cells per group. Figure 4: Confocal line-scan measurements of spontaneous calcium transients and caffeine-induced calcium release in SAN cells isolated from WT and DN-MCU mice. ( a ) Typical calcium transient images and spatially averaged traces in spontaneous beating SAN cells. ( b ) Typical caffeine-induced calcium release images and spatially averaged traces. ( c ) Summaries of spontaneous diastolic calcium release events and SR calcium content before and after ISO. Scatter graph of diastolic calcium events before and after ISO (upper panel). Bar graph of diastolic calcium release events before and after ISO (middle panel). Bar graph of SR calcium content determined by caffeine-evoked calcium release before and after ISO (lower panel). * P <0.05, ** P <0.01 versus control, # P <0.05 versus WT by Student’s t -test, n =11–21 cells per group. 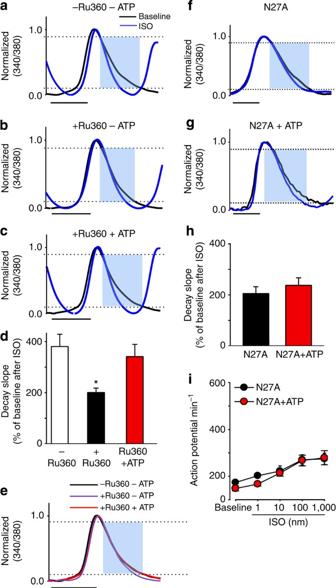Figure 5: ISO-induced acceleration of cytoplasmic Ca2+squestration is reduced by Ru360 but rescued by ATP. (a–c) Example averaged tracings show baseline (black) and ISO-stimulated (blue) intracellular Ca2+transients during spontaneous SAN cell activity measured under conditions as shown inFig. 1a–c. Ca2+transients were normalized to peak values for analysis of the decay phase. The decay phase of each tracing (marked by blue background), between the dashed lines marking 90–10% of peak values, shows rates of cytoplasmic Ca2+sequestration. Scale bar, 100 ms. (d) Summary data for the cytoplasmic Ca2+decay slope from 90% to 10% of the peak amplitude before and after ISO. *P<0.05 versus all other groups.n=5–10 per group, one-way analysis of variance. (e) Superimposed (baseline) traces froma–cshow that Ru360 or Ru360+ATP did not affect baseline Ca2+sequestration compared with control (−Ru360). Scale bar, 100 ms. (f–i) The PLN super-inhibitor N27A mutant slowed SAN cell rates and cytoplasmic Ca2+sequestration by a mechanism that was resistant to rescue by ATP dialysis. (f,g) Example tracings as in (a–c). Scale bar, 100 ms. (h) Summary data for the slope of the cytoplasmic Ca2+decay, as ind, NS between the groups,n=5–10 per group, unpaired Student‘st-test. (i) Summary dose–response data for AP rate responses to ISO in SAN cells from N27A transgenic mice with and without ATP dialysis. NS for all comparisons,n=5–10 per group, unpaired Student‘st-test. Error bars indicate s.e.m. Full size image Figure 5: ISO-induced acceleration of cytoplasmic Ca 2+ squestration is reduced by Ru360 but rescued by ATP. ( a – c ) Example averaged tracings show baseline (black) and ISO-stimulated (blue) intracellular Ca 2+ transients during spontaneous SAN cell activity measured under conditions as shown in Fig. 1a–c . Ca 2+ transients were normalized to peak values for analysis of the decay phase. The decay phase of each tracing (marked by blue background), between the dashed lines marking 90–10% of peak values, shows rates of cytoplasmic Ca 2+ sequestration. Scale bar, 100 ms. ( d ) Summary data for the cytoplasmic Ca 2+ decay slope from 90% to 10% of the peak amplitude before and after ISO. * P <0.05 versus all other groups. n =5–10 per group, one-way analysis of variance. ( e ) Superimposed (baseline) traces from a – c show that Ru360 or Ru360+ATP did not affect baseline Ca 2+ sequestration compared with control (−Ru360). Scale bar, 100 ms. ( f – i ) The PLN super-inhibitor N27A mutant slowed SAN cell rates and cytoplasmic Ca 2+ sequestration by a mechanism that was resistant to rescue by ATP dialysis. ( f , g ) Example tracings as in ( a – c ). Scale bar, 100 ms. ( h ) Summary data for the slope of the cytoplasmic Ca 2+ decay, as in d , NS between the groups, n =5–10 per group, unpaired Student‘s t -test. ( i ) Summary dose–response data for AP rate responses to ISO in SAN cells from N27A transgenic mice with and without ATP dialysis. NS for all comparisons, n =5–10 per group, unpaired Student‘s t -test. Error bars indicate s.e.m. Full size image MCU is not a global effector of pacemaker currents Because heart rate is responsive to multiple ionic currents [16] , we next asked if the MCU pathway affected the ATP and 3′-5′-cyclic adenosine monophosphate (cAMP)-dependent cell membrane ion channel (HCN4) inward current ( I f ) [23] an ionic current known to participate in SAN cell automaticity. We found that I f responses to ISO in isolated SAN cells were not reduced by Ru360 dialysis ( Fig. 6a,b ). The lack of effect of Ru360 on I f suggested that Ru360 did not reduce cAMP nor ATP availability globally in SAN cells below a threshold necessary to increase I f . To test this concept further, we measured the maximum diastolic cell membrane potential, which is primarily determined by activity of the Na + /K + ATPase [16] . MCU inhibition by Ru360 dialysis or by transgenic expression of DN-MCU did not affect the maximum diastolic membrane potential in isolated SAN cells ( Fig. 6c ). We also measured Ca V 1 L-type Ca 2+ current (I Ca ), an SAN cell membrane inward current enhanced by ISO through ATP-mediated phosphorylation [24] . Similar to our findings with I f , ISO-induced I Ca increases were not impaired by Ru360 ( Fig. 6d,e ). These findings were consistent with a model where selective loss of heart rate acceleration after ISO by Ru360 was primarily or exclusively related to actions on SERCA2a. 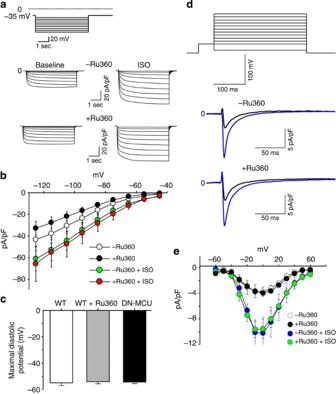Figure 6:IfandICaISO responses and maximum diastolic cell membrane potential are MCU independent. (a) RepresentativeIfcurrent recordings in response to voltage clamp commands (top panel) from an SAN cell without Ru360 (middle panel) and an Ru360-dialysed SAN cell (lower panel) before (left) and after ISO (right). (b) Summary current–voltage relationship forIffrom groups shown ina;n=4 SAN cells without Ru360 (−Ru360) andn=5 Ru360-dialysed cells (+Ru360). NS forIfcurrent density in Ru360-dialysed compared with SAN cells without Ru360 before and after ISO, unpaired Student‘st-test. (c) Maximum diastolic potential of spontaneous action potentials was not altered by MCU inhibition.n=12 per group. (d) RepresentativeICacurrent recordings in response to voltage clamp commands (top panel) from an SAN cell without Ru360 (-Ru360, middle panel) and an Ru360-dialysed SAN cell (+Ru360, lower panel) before (black trace) and after ISO (blue trace). (e) Summary current–voltage relationship forICafrom groups shown above.n=6–8 per group. NS forICacurrent density in +Ru360 compared with −Ru360 cells before and after ISO, unpaired Student‘st-test. Error bars indicate s.e.m. Figure 6: I f and I Ca ISO responses and maximum diastolic cell membrane potential are MCU independent. ( a ) Representative I f current recordings in response to voltage clamp commands (top panel) from an SAN cell without Ru360 (middle panel) and an Ru360-dialysed SAN cell (lower panel) before (left) and after ISO (right). ( b ) Summary current–voltage relationship for I f from groups shown in a ; n =4 SAN cells without Ru360 (−Ru360) and n =5 Ru360-dialysed cells (+Ru360). NS for I f current density in Ru360-dialysed compared with SAN cells without Ru360 before and after ISO, unpaired Student‘s t -test. ( c ) Maximum diastolic potential of spontaneous action potentials was not altered by MCU inhibition. n =12 per group. ( d ) Representative I Ca current recordings in response to voltage clamp commands (top panel) from an SAN cell without Ru360 (-Ru360, middle panel) and an Ru360-dialysed SAN cell (+Ru360, lower panel) before (black trace) and after ISO (blue trace). ( e ) Summary current–voltage relationship for I Ca from groups shown above. n =6–8 per group. NS for I Ca current density in +Ru360 compared with −Ru360 cells before and after ISO, unpaired Student‘s t -test. Error bars indicate s.e.m. Full size image MCU is required for ISO to increase NADH Mitochondrial Ca 2+ entry increases oxidative phosphorylation by enhancing the activity of key mitochondrial dehydrogenases to provide NADH/NADPH-reducing equivalents required for ATP synthesis [25] . This mechanism is activated when cellular Ca 2+ enters the inner mitochondrial membrane space from the cytosol through the MCU pathway [26] . We first asked whether mitochondrial Ca 2+ entry was critical for oxidative phosphorylation-dependent ATP synthesis in SAN pacemaker cells. We infected cultured mouse SAN cells with adenovirus encoding mt-pericam [27] , a circularly permutated Ca 2+ -sensitive fluorescent protein, to measure mitochondrial Ca 2+ concentration ([Ca 2+ ] mito ). The mt-pericam expression was localized to mitochondria in adenovirus infected SAN pacemaker cells, based on co-localization with MitoTracker Orange ( Fig. 7a ). ISO caused an increase in [Ca 2+ ] mito ( Fig. 7b ) that was prevented by dialysis of Ru360 ( Fig. 3b–d ). Mitochondrial Ca 2+ enhances ATP production by augmenting NADH, the primary electron donor for electron transport [28] . We next measured NADH fluorescence at baseline and after addition of ISO. ISO increased NADH fluorescence and this increase was prevented by Ru360 ( Fig. 8a,b , Supplementary Fig. 7a,b ) and in SAN cells with transgenic DN-MCU expression ( Supplementary Fig. 7c,d ), suggesting that ISO enhancement of NADH required MCU-mediated mitochondrial Ca 2+ entry. These data confirm the MCU-dependence of coupling between [Ca 2+ ] cyto and [Ca 2+ ] mito in SAN cells and show that the MCU provides critical metabolic support for SERCA2a activity and SR Ca 2+ loading. Together these data are consistent with a model where MCU-mediated enhancement of oxidative phosphorylation is a metabolic mechanism enabling the physiological fight or flight stress response in cardiac pacemaker cells ( Fig. 8c ). 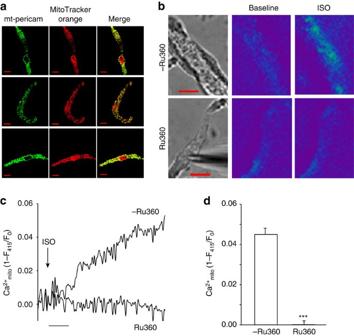Figure 7: ISO increases SAN cell mitochondrial Ca2+. (a) Adenovirus infected SAN cells expressing mt-pericam co-localized with MitoTracker (scale bar, 10 μm). (b) The mt-pericam fluorescence signal was increased by ISO (100 nM) stimulation and Ru360 dialysis prevented this increase (scale bar, 10 μm). (c) Example tracings show ISO increases in mitochondrial [Ca2+] ([Ca2+]mito) were prevented by Ru360 dialysis (scale bar, 100 s). (d) Summary data for [Ca2+]mitoresponses to ISO. ***P<0.001,n=14–15 per group, unpaired Student‘st-test. Error bars indicate s.e.m. Figure 7: ISO increases SAN cell mitochondrial Ca 2+ . ( a ) Adenovirus infected SAN cells expressing mt-pericam co-localized with MitoTracker (scale bar, 10 μm). ( b ) The mt-pericam fluorescence signal was increased by ISO (100 nM) stimulation and Ru360 dialysis prevented this increase (scale bar, 10 μm). ( c ) Example tracings show ISO increases in mitochondrial [Ca 2+ ] ([Ca 2+ ] mito ) were prevented by Ru360 dialysis (scale bar, 100 s). ( d ) Summary data for [Ca 2+ ] mito responses to ISO. *** P <0.001, n =14–15 per group, unpaired Student‘s t -test. Error bars indicate s.e.m. 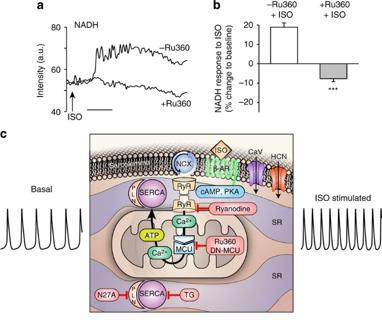Figure 8: Ru360 prevents ISO-stimulated increases in NADH. (a) Example of NADH fluorescence responses to ISO (100 nM) in control (–Ru360) and Ru360 dialysed SAN cells. Scale bar, 100 s. (b) Summary data for NADH fluorescence responses to ISO. ***P<0.001,n=7–18 per group, unpaired Student‘st-test. Error bars indicate s.e.m. (c) Proposed mechanism for MCU-enhancing SAN responses to ISO. β-AR, beta adrenergic receptor; CaV, voltage-dependent Ca2+channels; DN-MCU, dominant-negative MCU; HCN, hyperpolarization-activated cyclic nucleotide-gated channels; MCU, mitochondrial calcium uniporter; N27A, super-inhibitory phospholamban; NCX, Na+/Ca2+exchanger; PLN, phospholamban; SERCA, sarco/endoplasmic reticulum Ca2+-ATPase; SR, sarcoplasmic reticulum; TG, thapsigargin. Full size image Figure 8: Ru360 prevents ISO-stimulated increases in NADH. ( a ) Example of NADH fluorescence responses to ISO (100 nM) in control (–Ru360) and Ru360 dialysed SAN cells. Scale bar, 100 s. ( b ) Summary data for NADH fluorescence responses to ISO. *** P <0.001, n =7–18 per group, unpaired Student‘s t -test. Error bars indicate s.e.m. ( c ) Proposed mechanism for MCU-enhancing SAN responses to ISO. β-AR, beta adrenergic receptor; CaV, voltage-dependent Ca 2+ channels; DN-MCU, dominant-negative MCU; HCN, hyperpolarization-activated cyclic nucleotide-gated channels; MCU, mitochondrial calcium uniporter; N27A, super-inhibitory phospholamban; NCX, Na + /Ca 2+ exchanger; PLN, phospholamban; SERCA, sarco/endoplasmic reticulum Ca 2+ -ATPase; SR, sarcoplasmic reticulum; TG, thapsigargin. Full size image Our data provide new mechanistic understanding into the fight or flight response to physiological stress by showing that heart rate increases rely on the MCU in cardiac pacemaker cells. In contrast, basal rates do require SERCA activity but are independent of MCU, suggesting that availability of MCU-independent ATP production is sufficient to sustain heart rates in the absence of extreme physiological stress. Oxidative phosphorylation is enhanced by [Ca 2+ ] mito , which is required to generate ATP that fuels SERCA2a activity under extreme physiological stress. Our findings show that Ca 2+ homeostatic mechanisms in pacemaker cells form the framework for fight or flight heart rate increases but do not exclude additional modulation of heart rate by other Ca 2+ sensitive signals [29] , [30] or by Ca 2+ independent ionic currents [16] . The MCU metabolic pathway appears optimized to generate heart rate increases during episodes of high energy demand that are signalled by catecholamines. Our data are consistent with earlier work showing that mitochondrial Ca 2+ is required to optimize refilling of intracellular Ca 2+ stores by SERCA2a [31] and where ATP dialysis (3 mM) recovered Ca 2+ sequestration by intracellular stores after the addition of mitochondrial toxins [32] . Our findings provide insight into recent work showing MCU knockout selectively impairs high workload activity in striated muscle [33] . However, our data show that basal pacemaker cell activity is uncoupled from MCU-dependent ATP production. Because the relationship between MCU and SERCA2a in pacemaker cells appears purposed to selectively enable heart rate acceleration, future therapies targeting MCU or SERCA2a in pacemaker cells could provide a means to fine tune heart rates by preventing excessive heart rates without reducing resting heart rates. All the experiments were carried out in accordance with the guidelines of Institutional Animal Care and Use Committee (PHS Animal Welfare Assurance, A3021-01). SAN cell isolation and electrophysiological recordings Isolation of single SAN cells from mice was performed according to previously published methods [29] , [34] with minor modifications. Mice (6–8 weeks, females and males) were administered an intraperitoneal injection of avertin (20 μl g −1 ) and monitored until unresponsive. The heart was excised and placed into Tyrode’s solution (35 °C), consisting of (mM) 140.0 NaCl, 5.0 HEPES, 5.5 glucose, 5.4 KCl, 1.8 CaCl 2 and 1.0 MgCl 2 . The pH was adjusted to 7.4 with NaOH. The SAN region, delimited by the crista terminalis, atrial septum and orifice of superior vena cava, was dissected free from the heart. The SAN was cut into smaller pieces, which were transferred and rinsed in a solution containing (mM) 140.0 NaCl, 5.0 HEPES, 5.5 glucose, 5.4 KCl, 0.2 CaCl 2 , 0.5 MgCl 2 , 1.2 KH 2 PO 4 , 50.0 taurine and 1.0 mg ml −1 bovine serum albumin, with pH adjusted to 7.4 using NaOH. SAN tissue pieces were digested in 5 ml of solution containing collagenase type I, elastase (Worthington) and protease type XIV (Sigma) for 20–30 min. The tissue was transferred to 10 ml of Kraft–Bruhe medium containing (mM) 100.0 potassium glutamate, 5.0 HEPES, 20.0 glucose, 25.0 KCl, 10.0 potassium aspartate, 2.0 MgSO 4 , 10.0 KH 2 PO 4 , 20.0 taurine, 5.0 creatine, 0.5 EGTA and 1.0 mg ml −1 bovine serum albumin, with pH adjusted to 7.2 using KOH. The tissue was agitated using a glass pipette for 10 min. The cells were stored at 4 °C and studied within 7 h. SAN cells were placed in Tyrode’s solution at 36±0.5 °C. SAN cells were identified by their characteristic morphology (spindle or spider shape) and spontaneous activity in all single-cell experiments. SAN cells were also identified electrophysiologically by typical spontaneous action potentials with slow depolarizing phase 4 and the hyperpolarization-activated current ( I f ) in electrophysiological experiments. Spontaneous action potentials and I f were recorded using the perforated (amphotericin B or β-escin) patch-clamp technique [35] on single SAN cell at 36±0.5 °C in Tyrode’s solution (0.5 mM BaCl 2 was added to the bath solution when recording I f [36] , [37] ). The pipette was filled with (mM) 130.0 potassium aspartate, 10.0 NaCl, 10.0 HEPES, 0.04 CaCl 2 , amphotericin B 240 μg ml −1 with pH adjusted to 7.2 with KOH. SAN cells with stable action potentials lasting at least 5 min were included in the experiments. β-escin 25 μM was substituted for amphotericin B to allow dialysis of Ru360 or ATP. When recording I f , membrane potential was held at −35 mV, the voltage steps were applied for 5 s ranging from −125 mV to −45 mV in 10 mV increments or vice versa [38] . I Ca was measured using the perforated patch technique at 36±0.5 °C as previously described [29] . I Ca was confirmed by its sensitivity to nifedipine 5 μM. Depolarizing voltage pulses (300 ms in duration) to various potentials (−60 mV to 60 mV in 10 mV step) were applied after 50 ms at −40 mV to inactivate I Na from a holding potential of −70 mV. The pipette solution comprised (mM): 120.0 CsCl, 10.0 EGTA, 10.0 HEPES, 10.0 tetraethylammonium chloride, 5.0 phosphocreatine, 3.0 CaCl 2 , 1.0 MgATP, 1.0 NaGTP and the pH was adjusted to 7.2 with 1.0 N CsOH. The bath (extracellular) solution comprised (mM): 137.0 NaCl, 10.0 HEPES, 10.0 glucose, 1.8 CaCl 2 , 0.5 MgCl 2 , 25.0 CsCl, pH was adjusted to 7.4 with NaOH. Viral infection with 5mt-pericam/eGFP and DN-MCU Freshly isolated mouse (6–8 weeks, females and males) SAN tissue was cut into small pieces and put into 35 mm tissue culture plates with DMEM. Fresh medium containing Ad-eGFP, Ad-5mt-pericam or Ad-DN-MCU was added to the plates at a multiplicity of infection of 100. Ad-5mt-pericam and Ad-DN-MCU were generated as follows: Ratiometric-Pericam-mt [27] was first subcloned into pacAd5CMV-mcs-KN (University of Iowa Gene Transfer Vector Core) using HindIII and EcoRI. As the localization of this Pericam with a single Cox4 targeting sequence was not exclusive to mitochondria, four additional mitochondrial targeting sequences were added to the amino terminus. Two tandem Cox8a targeting repeat units from the pcDNA3-D4cpv vector [39] were subcloned via HindIII into pacAd5CMV-ratiometric-Pericam-mt. Colonies were screened to identify clones that contained four tandem Cox8a inserts and confirmed via sequencing. For Ad-DN-MCU containing a carboxy (C)-terminal Myc tag, human MCU cDNA clone (GenBank accession code BC034235) was first obtained from the I.M.A.G.E consortium (ID: 5296557) and subcloned into pAd5CMVmcsIRESeGFP (University of Iowa Gene Transfer Vector Core, Iowa City, IA, USA) by PCR using Phusion DNA Polymerase (New England Biolabs) and the GeneArt Seamless Cloning and Assembly Kit (Life Technologies). PCR primers amplifying Myc-tagged MCU were: forward 5′- ATAAGCTTATGGCGGCCGCCGCAGGTAGATCG -3′, reverse 5′- CTACAGGTCTTCTTCGCTAATCAGTTTCTGTTCATCTTTTTCACCAATTTGTCGGAG -3′, and pAd5CMVmcsIRESeGFP: forward 5′- GAAGAAGACCTGTAGGATATCGAATTCCTGCAGCCC -3′, reverse 5′- GCCGCCATAAGCTTATCGATACCGTCGACCTC -3′. Dominant-negative mutations in MCU that inhibit Ca 2+ conductance (D260Q, E263Q) [7] , [8] were generated with Agilent’s QuikChange site-directed mutagenesis kit. Positive clones were confirmed by DNA sequencing. Adenoviruses expressing of 5mt-Pericam and DN-MCU-myc were generated by the University of Iowa Gene Transfer Vector Core. Expression of the recombinant ratio-5mt-pericam and DN-MCU in SAN cells was detected by GFP fluorescence. Recombinant adenovirus that expresses eGFP only (Ad-eGFP) was used as a control. NADH and mitochondrial Ca 2+ measurements The autofluorescence of endogenous NADH, which derives primarily from mitochondria [40] , [41] , was measured as described [41] . In brief, NADH was excited at 350 nm (AT350/50X, Chroma) and fluorescence was recorded at 460 nm (ET460/50m and T400LP, Chroma). We normalized NADH level with FCCP as 0%, Rotenone-induced NADH change as 100%. The baseline level of NADH was 22%±3 ( n =15) of the rotenone-induced maximal value. Mt-pericam, a mitochondrial matrix-targeted, circularly-permuted green fluorescent protein fused to calmodulin and its target peptide M13 (ref. 27 ). Pericam emission at 535 nm due to excitation at 415 nm reports changes in Ca 2+ (ref. 42 ). We used 5 mt-pericam to measure Ca 2+ mito in isolated, cultured SAN cells. The mitochondrial Ca 2+ level was monitored in cells transiently expressing the 5 mt-pericam protein at excitation wavelengths of 415 nm, presented as 1−F/F 0 (Ca 2+ mito ) (refs 42 , 43 , 44 ), and the emission collected using a 535-nm band-pass filter. Intracellular Ca 2+ transients Cytosolic Ca 2+ levels were recorded from Fura-2–loaded cells, excited at wavelengths of 340 and 380 nm, and imaged with a 510-nm long-pass filter. Single isolated SAN cells were loaded with 0.1 μM Fura-2 AM for 20 min, and then perfused for 20 min to de-esterify the Fura-2 AM in normal Tyrode’s solution. After placement on a recording chamber, the cells were perfused in normal Tyrode’s solution at 36 °C±0.5. Spindle-shaped, spontaneously beating cells were chosen for the experiments. Action potential recording was performed simultaneously. SAN gene painting SAN painting was performed as previously described [14] , [45] . Briefly, Poloxamer 407 (Spectrum), trypsin (Sigma) and collagenase, type II (Worthington) mixture was made with 40% Poloxamer, 1% trypsin and 0.25% collagenase in PBS, and then added to an equal volume of recombinant adenovirus expressing cDNA for the gene(s) of interest (DN-MCU-IRES GFP vs eGFP) in solution. This mixture was liquid in consistency at 4 °C but gelled at 37 °C. Mice (6–7 weeks, females and males) were anaesthetized using ketamine/xylazine (87.5/12.5 mg kg −1 , respectively), intubated and ventilated. The junction of the superior vena cava and right atrium was visualized through a small incision in the second intercostal space. The gel was applied to the posterior surface of the junction of the superior vena cava and right atrium with a fine brush. The intercostal muscles, pectoralis major and minor and the skin incision were closed using 6/0 silk and the mice were allowed to recover. Ex vivo Langendorff-perfused heart rate measurements ECG recording from Langendorff-perfused hearts was performed as described [29] . Briefly, excised hearts from 7 to 9-week female and male mice were rapidly mounted on a modified Langendorff apparatus (HSE-HA perfusion systems, Harvard Apparatus, Holliston, Mass) for retrograde aortic perfusion at a constant pressure of 80 mm Hg with oxygenated (95% O 2 , 5% CO 2 ) Krebs–Henseleit solution consisting of (mM) 25.0 NaHCO 3 , 118.5 NaCl, 4.0 KCl, 1.2 MgSO 4 , 1.2 NaH 2 PO 4 , 1.5 CaCl 2 and 11.2 glucose, with pH equilibrated to 7.4. Each perfused heart was immersed in a water-jacketed bath and was maintained at 36 °C. ECG measurements from the intact heart were continuously recorded with Ag + -AgCl electrodes, which were positioned around the heart in an approximate Einthoven configuration. After the heart was allowed to stabilize for 15 min, different concentrations of isoproterenol were added to the perfusate. Immunofluorescence staining The SAN area was dissected from freshly isolated hearts for comparing transgenic DN-MCU mice with WT or from Langendorff perfused hearts for localizing SAN gene painted tissue. The SAN tissue was imbedded in OCT tissue freezing media and cooled over liquid nitrogen before being stored at −80 °C. 10 μM serial sections were taken through the tissue. All sections were slowly brought from −20 °C to room temperature in 4% paraformaldehyde. Sections were washed with ice cold PBS, permeabilized (0.1% Triton X-100, 0.1% sodium citrate in PBS) and blocked (3% fish gelatin, 2 mg ml −1 BSA, 0.1% Triton X-100 in PBS). HCN 4 (Abcam) (1:200) and Myc epitope tag (Rockland) (1:200) antibodies were incubated with samples overnight at 4 °C. Samples were washed in blocking buffer and fluorophore conjugated secondary antibodies (1:500) were incubated overnight. Gene painted sections were treated with DAPI and imaged on an EVOS FL Auto microscope. DN-MCU transgenic samples and WT sections were images on a confocal microscope (Zeiss). Calcium green mitochondrial Ca 2+ uptake assays We measured mitochondrial Ca 2+ uptake using permeabilized HEK cells as previously described [46] , [47] . Briefly, cells were grown in DMEM, with 10% FBS and 1% of Penicillin/Streptomycin. At 80% confluence cells were infected with DN- MCU adenovirus at MOI 10. Cells were harvested after 24 h incubation and placed into a 96 well plate. Each well was loaded with 1 million cells in respiratory buffer containing 125.0 mM KCl, 2.0 mM K 2 HPO 4 , 20.0 mM HEPES, 5.0 mM glutamate, 5.0 mM malate, 0.005% saponin, and 5 μM thapsigargin. 5 μM Ca 2+ was injected at 3 min intervals. Fluorescence was measured using a Tecan plate reader. Adult cardiac myocytes were isolated from 6- to 8-week-old wild-type or DN-MCU TG mice using a previously described isolation procedure [46] . A total of 50 nM Blebbistatin was included in the myocyte buffer to prevent cellular contraction. Fluorescence intensity was measured from 50,000 cardiac myocytes per well. Then, 100 μM Ca 2+ was injected at 3-min intervals for myocyte experiments. DN-MCU overexpressing mice The inter-membrane D 260 IME 263 amino-acid motif of human MCU was mutated to the dominant-negative (DN) form [8] , QIMQ, by replacing the nucleotide sequence, 5′- gacatcatggag -3′ with 5′- cagatcatgcag -3′ using site-directed mutagenesis (agilent.com). The resulting DN-MCU DNA product was amplified by PCR with Phusion DNA polymerase using a forward primer containing a SalI restriction site (5′- ACCAACGTCGACATGGCGGCCGCCGCAGGTAG -3′) and reverse primer containing a C-terminal myc epitope tag sequence and HindIII restriction site (5′- GAACGCAAGCTTCCTACAGGTCTTCTTCGCTAATCAGTTTCTGTTCATCTTTTTCACCAATTTGTCGGAG -3′). PCR products were digested and ligated into SalI and HindIII digested pBS-αMHC-script-hGH vector and positive clones confirmed by sequencing. Mouse embryonic stem cells were injected with the linearized DNA (digested with NotI) in the University of Iowa Transgenic Mouse Core Facility and implanted into pseudo-pregnant females to generate B6XSJL F1 mice. Insertion of the transgene into the mouse genome was confirmed by PCR analysis (not shown) using the forward primer, 5′- CCCACACCAGAAATGACAGACAGAT -3′ and reverse primer, 5′- AGAGGAGCAGCAGGAGCGATCTA -3′, producing a product of 200 bases. Mice were backcrossed to F4 generation or greater into the CD1 background. Transgenic and control mice of either gender were killed at the age of 2–3 months. Western blots for detecting phospholamban Heart lysates were prepared from flash-frozen mouse right atria from 6- to 8-week-old female and male mice. Mice were injected with ISO (0.4 mg kg −1 ) 10 min before harvesting the right atrium and western blotting was performed with a SDS–polyacrylamide gel electrophoresis (SDS–PAGE) electrophoresis system as described [29] . Briefly, 30 μg protein samples were size-fractionated on SDS–PAGE, and then transferred to polyvinylidene difluoride membranes. The membranes were probed with anti-pSer16-PLN (1:5,000), anti-pThr17-PLN (1:5,000) (from Badrilla Ltd., Leeds, UK) at room temperature for 4 h. Then membranes were incubated with Alexa-Fluor680-conjugated anti-mouse (Invitrogen Molecular Probes, Carlsbad, CA, USA) and/or IR800Dyeconjugated anti-rabbit fluorescent secondary antibodies (Rockland Immunochemicals, Gilbertsville, PA, USA) and scanned on an Odyssey infrared scanner (Li-Cor, Lincoln, NE, USA). Integrated densities of protein bands were measured using ImageJ Data Acquisition Software (National Institute of Health, Bethesda, MD, USA). Uncropped scans of all western blot images are available in the SI. Western blots for detecting MYC-tagged DN-MCU Heart, liver and skeletal muscle tissues were harvested and flash frozen. Samples were homogenized in RIPA buffer (10 mM Tris-Cl, pH8.0, 1 mM EDTA, 1% Triton X-100, 0.1% sodium deoxycholate, 0.1% SDS, 140 mM NaCl), containing protease and phosphatase inhibitors with antioxidant. Twenty micrograms of protein were fractionated on NuPAGE (Invitrogen) 4–12% SDS–PAGE gels and transferred overnight to polyvinylidene difluoride membranes (Bio-Rad). Nonspecific binding was blocked with 10% w/v non-fat milk powder in TBS-T (50 mM Tris-HCl, pH 7.6, 150 mM NaCl, 27 mM KCl and 0.25% Tween-20). The membranes were probed with anti-MYC (1:1,000) (Rockland Immunochemicals, Gilbertsville, PA, USA) at room temperature for 2 h. Then membranes were incubated with anti-rabbit HRP-conjugated secondary antibody (1:5,000). Protein bands were visualized using ECL reagent (Lumi-Light, Roche). Correct loading was confirmed with Coomassie staining of membranes. Uncropped scans of all western blot images are available in the SI. Mouse surface electrocardiograms Mouse surface electrocardiogram (ECG) tracings were acquired as described [48] . Before the ECG acquisition 6- to 8-week-old female and male mice were pre-anaesthetized with 2% isoflurane in 1l oxygen per minute (Isotec100 Series, Isoflurane Vaporizer, Harvard Apparatus, Holliston, USA). Mice were placed in a supine position on a heated ECG pad (Mousepad, THM 100, Indus Intruments, Webster, USA), and the limbs were attached to the pad electrodes using a tape to obtain ECG lead II. Anaesthesia was maintained via facemask by continuous isoflurane ventilation as described above. The body temperature was continuously monitored using a rectal probe and sustained within 36–37 °C. To obtain a baseline ECG, animals were allowed to rest for 5 min after being positioned on the pad. Thereafter isoproterenol (10 μg kg −1 ) was injected intraperitoneally. ECG acquisition was performed continuously using a multichannel amplifier and data acquisition system (Powerlab 16/30, AD Instruments, Colorado Springs, USA) converting the signal into digital for a further data analysis (Labchart Pro software, version 7, AD Instruments, Colorado Springs, USA). Laser scanning confocal imaging of single SAN cells Laser scanning confocal imaging of single SAN cells were performed as described [49] . Mouse SAN cells isolated from WT or DN-MCU mice were loaded with Fluo-4 AM (5 μM) for 20 min at room temperature. After 20 min of de-esterification, the cells were placed in a recording chamber and perfused with normal Tyrode solution (1.8 mM Ca 2+ ) at 36±1 °C (Temperature Controller, TC2BIP, Cell MicroControls). Spindle-shaped, active spontaneously beating cells were chosen for the experiments. Confocal Ca 2+ imaging was performed in line-scan mode with a laser scanning confocal microscope (LSM 510, Carl Zeiss) equipped with a numerical aperture (NA) 1.35, × 63 lenses. Images of spontaneously beating Ca 2+ transients and caffeine-induced Ca 2+ transients (SR Ca 2+ contents) were acquired at a sampling rate of 1.93 ms per line along the longitudinal axis of the cells. SR Ca 2+ content was determined by measuring the amplitude of Ca 2+ release induced by local delivery of 20 mM caffeine. All digital images were processed with IDL 6.0 program (Research System Inc). Electrocardiographic telemetry Surgical implantation of ECG telemeters was performed as described [29] . In brief, 8- to 10–week-old female and male mice were anaesthetized with ketamine/xylazine (87.5/12.5 mg kg −1 ), and an ECG transmitter (DSI model Ta10EA-F20) was implanted in the abdominal cavity. The leads were placed subcutaneously in a lead I configuration. Experiments were performed after a 5-day recovery period. ECG and activity were recorded for 72 h from undisturbed mice at a sampling rate of 1 kHz. Heart rate and activity were calculated from serial 1-min averages. On the fourth day, there was a 1-h baseline ECG recorded before ISO injection followed by an ISO injection and an additional 1-h recording epoch. On the fifth day, we repeated this protocol with another dose of ISO. The last dose of ISO was given on the sixth day. The heart rate in response to ISO was calculated from serial 10-s averages. Echocardiography Transthoracic echocardiography was performed as previously described [50] . Unanesthetized, sedated mice were used for echocardiography. A 30-MHz linear array transducer was applied to the chest to obtain cardiac images. The transducer was coupled to a Vevo 2100 imager (FUJIFILM Visual Sonics, Toronto, Canada). Images of the short and long axis were obtained with a frame rate of ~180–250 hertz. All image analysis was performed offline using Vevo 2100 analysis software (Version 1.5). ATP measurements The 6- to 8-week-old littermate mice were killed. Atria were rapidly harvested and flash frozen in liquid nitrogen. Atria were homogenized, sonicated and centrifuged at 10,000 g . The supernatants were collected and a luciferase assay (Invitrogen, ATP Determination Kit A22066) was used to detect ATP. Samples were measured in triplicate on a Femtomaster FB 12 luminometer (Zylux). Quantitative RT PCR RNA was isolated using Trizol reagent (Invitrogen) and purified using a RNeasy MinElute Cleanup Kit (Qiagen). RNA concentrations were measured using a Nanodrop 2000 spectrophotometer (Thermo Scientific). iScript cDNA Synthesis Kit (Bio-Rad) was used to generate cDNA from RNA using oligo(dT) primers. Validated PCR primers (Bio-Rad) were used for qRT PCR on a StepOnePlus Real-Time PCR system (Applied Biosystems). Transcript levels were quantified by the ΔΔCt method. Statistical analysis Data are presented as mean±s.e.m., unless otherwise noted. Statistical analysis was performed either with one-way analysis of variance or an unpaired or paired Student’s t -test, as appropriate. The Holm–Sidak test was used for post hoc comparisons after analysis of variance. Analyses were performed with Sigmaplot or Sigmastat (Systat Software, Inc. San Jose, CA 95110, USA). The null hypothesis was rejected for a P <0.05. How to cite this article: Wu, Y. et al . The mitochondrial uniporter controls fight or flight heart rate increases. Nat. Commun. 6:6081 doi: 10.1038/ncomms7081 (2015).